Microscopic magnetic stimulation of neural tissue Electrical stimulation is currently used to treat a wide range of cardiovascular, sensory and neurological diseases. Despite its success, there are significant limitations to its application, including incompatibility with magnetic resonance imaging, limited control of electric fields and decreased performance associated with tissue inflammation. Magnetic stimulation overcomes these limitations but existing devices (that is, transcranial magnetic stimulation) are large, reducing their translation to chronic applications. In addition, existing devices are not effective for deeper, sub-cortical targets. Here we demonstrate that sub-millimeter coils can activate neuronal tissue. Interestingly, the results of both modelling and physiological experiments suggest that different spatial orientations of the coils relative to the neuronal tissue can be used to generate specific neural responses. These results raise the possibility that micro-magnetic stimulation coils, small enough to be implanted within the brain parenchyma, may prove to be an effective alternative to existing stimulation devices. Electrical stimulation of excitable tissue is a rapidly expanding viable therapeutic strategy for treating human disorders. For example, deep brain stimulation (DBS) has been successful in the treatment of movement disorders such as Parkinson's disease, dystonia and essential tremor, and clinical trials are currently underway to examine its efficacy for the treatment of additional neurological and psychiatric diseases including epilepsy, major depression and obsessive-compulsive disorder [1] , [2] . Electrical stimulation of the muscle has a long therapeutic history; the most notable example is the use of cardiac pacemakers for the treatment of conduction and arrhythmia disorders of the heart. There has also been success in using cochlear implants to restore auditory function [3] , and considerable efforts are underway to develop limb [4] and visual prostheses [5] , [6] , [7] . Despite the successes of direct electrical stimulation, its implementation comes with some technical and biological limitations. For example, magnetic resonance imaging (MRI) examination of DBS patients can result in neurological damage because of excessive heating at the stimulating electrode tip [8] . In these patients, heating is induced by MRI-generated radio-frequency waves that interact with the conductive leads to generate induced currents (known as the 'antenna effect'), which result in the loss of energy in the form of heat [9] . In addition, safety concerns have been raised for pacemakers owing to the reported changes in cardiac pacing after MRI that may also be related to contact tip heating [10] . Another challenge with direct electrical stimulation is that the therapeutic effects can be altered by inflammatory and immune reactions of the tissue in response to direct contact with the stimulating electrode [11] . For example, glial scarring around the stimulating electrode will eventually increase electrode impedance and stimulation thresholds [12] . The use of transcranial magnetic stimulation (TMS) for the diagnosis and treatment of neurological disorders has been studied for over two decades [13] , [14] . TMS uses hand-held coils positioned over the scalp to generate very large time-varying magnetic fields (for example, >1T), which induce currents that modulate neural activity. Experimental evidence suggests that TMS has therapeutic benefits for treating a number of neurological disorders, such as major depression and stroke [15] . However, employing TMS as a standard medical therapy has several limitations. TMS devices must be large to create magnetic fields strong enough to activate neural tissue across large distances. As a result, TMS therapy requires the patient to be in the clinic for long durations, which is both costly and inconvenient. In addition, TMS generally targets superficial cortical regions, as deeper targets, such as the basal ganglia, are beyond the range of current technology. Moreover, accurate focus of specific neuronal targets is difficult [16] as spatial control with existing devices is limited. Part of the success of electrical stimulation can be attributed to the array of relatively small electrodes, each capable of independently eliciting activity that is restricted to a focal region of tissue. This raises the question of whether a smaller magnetic device would be able to overcome some of the limitations that make TMS inherently unsuitable for chronic prosthetic applications. Electric currents flowing in these microcoils would presumably generate time-varying magnetic fields, similar to TMS, which would induce electric currents in a focal area. Recent work suggests that coils smaller than those used in conventional TMS devices can elicit neuronal responses [17] but such coils are still too large to be surgically implanted and it is not known whether sub-millimeter coils can in fact elicit neuronal responses. Micromagnetic stimulation (μMS) would have several advantages over conventional electrical stimulation. For example, microcoils are likely to be MRI compatible (when turned off) as the μMS coils are electrically isolated from the adjacent tissue, thus limiting the amount of heat induction. In addition, microscopic coils may be placed in close proximity to the tissue, potentially improving the spatial control of the elicited activity. Finally, these coils can be encapsulated with a wide range of biocompatible materials (for example, parylene [18] and liquid crystal polymer [19] , [20] ), which may help to reduce inflammation. To explore whether such small coils could indeed evoke neural activity, we used a combination of computational modelling and electrophysiological experiments. We first created a computational finite element method (FEM) model that allowed us to study the magnetic fields arising from μMS as well as the electric fields they induced. The model suggests that such fields would be sufficient to elicit neuronal activity. We confirmed this by recording from rabbit retinal ganglion cells while stimulating with the small coils and found that μMS does induce neural activity. Both the orientation of the coil and the magnitude of the stimulation parameters influenced the neuronal response, and a wide range of responses could be generated. Although further testing is required, our findings raise the possibility that μMS may be a suitable alternative to existing electric stimulation devices. Small coils induce sizable electric fields The theoretical equations governing the magnetic and electric fields that arise from current flowing through a coil are well established, but the fields that arise from sub-millimeter coils implanted in biological tissue, specifically, their ability to elicit neural activity, have not been previously explored. Magnetic field pulses induce a circulating electric field in the tissue owing to Faraday's law, expressed in one of the four Maxwell equations. Similarly to a boat in a whirlpool, the circulating electric fields ( E ) generate currents that tend to follow a circular path in conductors and depend on how quickly the magnetic fields ( B ) generated by the μMS change over time. The induced E values were estimated with the FEM by solving the set of Maxwell equations simplified by the magnetostatic assumption that all magnetic fields are switching on timescales of microseconds or slower [21] , as in the electrophysiology experiments. The FEM calculations were performed to determine whether microscopic coils used in the electrophysiology experiments could generate large enough E to evoke action potentials in neuronal tissue. The geometry consisted of a cylindrical container of 3 mm radius and 3 mm height, which enclosed different objects: a physiological solution, a quartz core surrounded by the copper solenoid, and top/bottom copper cylindrical terminals. The FEM calculations were performed on the model of a cylindrical inductor/coil with a 500-μm radius, a height of 1 mm and 21 turns ( Fig. 1 ), positioned inside a uniform volume conductor representing the saline solution or the retinal tissue with similar electrical characteristics. Given that the FEM simulations were in cylindrical two-dimensional coordinates, the coil can only be represented as a cylinder; the coil used in the simulations approximates the rectangular passive component structure of the actual inductor used in the electrophysiological experiments ( Fig. 2 ). The boundary conditions at the external surfaces of the cylindrical container were set to magnetic insulation (the magnetic field strength was set to zero). The FEM solution consisted of values in and around the cylindrical inductor of electric (V) and magnetic ( A ) potentials, which were used to calculate the induced E (Methods). 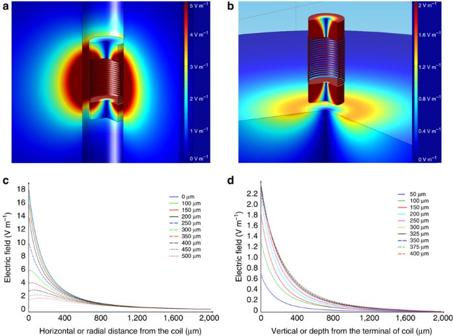Figure 1: The FEM simulations. (a) Three-dimensional distribution of the electric field around the coil starting at 100 μm from the edge of the device. (b) Three-dimensional distribution of the electric field starting at 100 μm below the terminal of the coil. (c) Plot of the radial distribution of the electric field from different elevations. Legend shows the different elevations from coil-center. (d) Plot of the axial distribution of the electric field from different radial distances from the axis of the device. Legend shows the different radial distances from coil-center. Figure 1: The FEM simulations. ( a ) Three-dimensional distribution of the electric field around the coil starting at 100 μm from the edge of the device. ( b ) Three-dimensional distribution of the electric field starting at 100 μm below the terminal of the coil. ( c ) Plot of the radial distribution of the electric field from different elevations. Legend shows the different elevations from coil-center. ( d ) Plot of the axial distribution of the electric field from different radial distances from the axis of the device. Legend shows the different radial distances from coil-center. 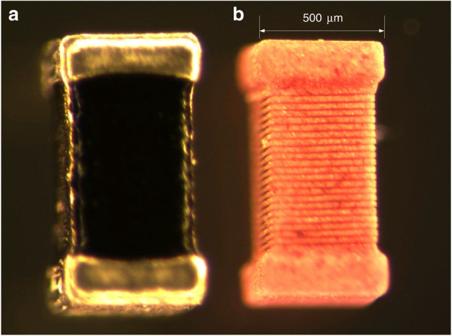Figure 2: Structure of the inductor. (a) Image of the inductor used in the electrophysiological experiments. (b) The outer layer of the inductor was chemically dissolved to expose the structure of the underlying solenoid. Full size image Figure 2: Structure of the inductor. ( a ) Image of the inductor used in the electrophysiological experiments. ( b ) The outer layer of the inductor was chemically dissolved to expose the structure of the underlying solenoid. Full size image When the long axis of the coil was oriented in parallel to the retinal surface ( Fig. 3a ), the maximum value of the strength of E was ~6 V m −1 at a distance of 200 μm from the edge of the dielectric (300 μm from the edge of the coil) ( Fig. 1a,c ); this distance was similar to that used in the electrophysiological experiments. These values are comparable to the 10 V m −1 thresholds for neuronal activation measured by Chan and Nicholson [22] . The strength of induced electric fields was attenuated nonlinearly with increased distance from the coil ( Fig. 1c ). The maximum values of the induced electric field ( Fig. 1b,d ) were much weaker when the coil was in perpendicular orientation ( Fig. 3b ) and were approximately 1 V m −1 at a distance of 200 μm (300 μm from the edge of the coil). Similar to the parallel orientation, the strength of the electric field decreased nonlinearly with distance when the coil was oriented perpendicular to the retinal surface ( Fig. 1d ). 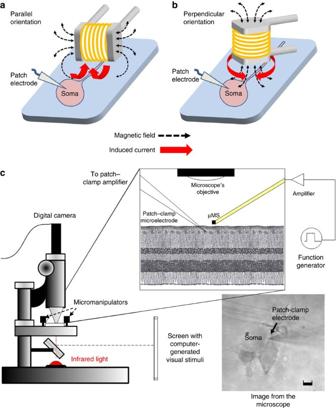Figure 3: Experimental setup of the micro magnetic stimulation of retinal neurons. (a,b) The two different stimulation-coil orientations that were tested: parallel (a) and perpendicular (b) refer to the relationship between the main axis of the coil and the retinal surface. (c) The retinal preparation was extracted and placed in a small recording chamber with the ganglion cell side facing up. Stimulation was delivered by a small coil located ~300 μm above the ganglion cell and responses were recorded via cell-attached patch–clamp electrodes positioned on the ganglion cell surface. The retina was illuminated via an infrared source and observed via a digital camera (Scale bar, 5 μm). A computer-controlled screen was used to project visual stimuli onto the retina. Figure 3: Experimental setup of the micro magnetic stimulation of retinal neurons. ( a , b ) The two different stimulation-coil orientations that were tested: parallel ( a ) and perpendicular ( b ) refer to the relationship between the main axis of the coil and the retinal surface. ( c ) The retinal preparation was extracted and placed in a small recording chamber with the ganglion cell side facing up. Stimulation was delivered by a small coil located ~300 μm above the ganglion cell and responses were recorded via cell-attached patch–clamp electrodes positioned on the ganglion cell surface. The retina was illuminated via an infrared source and observed via a digital camera (Scale bar, 5 μm). A computer-controlled screen was used to project visual stimuli onto the retina. Full size image In general, the threshold to stimulation depends on the so-called strength–duration curve [23] , which is not well understood for magnetic stimulation. Therefore, we could, in principle, increase the duration (5 μs) of the induced electric field by extending the duration of the rising or falling current in the μMS coils, as we can only induce an E field by generating a time-varying B field in the μMS coils. However, we are limited by the peak current (~±10A) before the coil is damaged. According to our experience, the copper traces used in our coils may carry a 6.6×10 9 A m −2 current density (DC) for 5–6 μs pulses before melting occurs, a value in line with the maximum current density used in TMS [24] . Finally, we could increase the strength of the induced E field by increasing the slope of the current pulse in the coils (even though, our amplifier was limited to 8×10 6 V s −1 ), but this would reduce the pulse length because we are limited by the maximum current in the coil as discussed previously. μMS activates retinal neurons To confirm that neurons could in fact be activated by μMS, we ran a series of electrophysiological experiments that measured the response of retinal ganglion cells to stimulation from a small, commercially available magnetic coil ( Fig. 2 ) that was assembled into a custom μMS device (Methods). The ability of coils that are small enough to be implanted sub-cortically to activate neuronal tissue had not been evaluated previously. Experimental methodology closely followed procedures, used previously, to measure responses of similar cells to electric stimulation [25] , [26] . The extracted retina was positioned ganglion cell side up ( Fig. 3c ) in a small chamber (~1 ml) and perfused with oxygenated Ames medium. Patch–clamp electrodes were positioned on the surface of the soma of targeted ganglion cells (cell-attached configuration) to detect action potentials elicited in response to magnetic stimulation. Before the onset of μMS testing, responses to full-field flashes of light were measured to ensure viability of each targeted ganglion cell; only those cells that generated robust light responses were used for subsequent μMS stimulation. All cells that generated spiking in response to light stimuli also generated spikes in response to μMS. The results below are derived from recordings in 12 ganglion cells (6 different retinas). Microcoils were positioned ~300 μm above the inner surface of the retina (Methods) in one of two configurations: the long axis of the coil was oriented either parallel ( Fig. 3a ) or perpendicular ( Fig. 3b ) to the surface of the retina. The coils were coated with a biocompatible high-strength insulator, and impedance was tested at the beginning and end of each experiment to eliminate the possibility that responses were mediated by a leakage of current from the wire into the retinal preparation (Methods). Consistent with the modelling results (above), action potentials were elicited in response to μMS ( Fig. 4 ). With the axis of the coil oriented parallel to the retinal surface, single μMS pulses elicited complex responses that consisted of a prolonged stimulus artefact ( Fig. 4a , duration of ~20 ms) followed by a series of biphasic waveforms. The amplitude and kinetics of individual biphasic waveforms were nearly identical to that of action potentials elicited in response to light stimuli ( Fig. 4b ), strongly suggesting that the biphasic waveforms were in fact action potentials. There were slight variations in the number and/or latency of elicited spikes from trial to trial ( Fig. 4a , each row is a separate trial from the same cell), although the general features of the response were consistent across trials ( Fig. 4c ). Similar responses were seen in all six cells for which the coil was oriented parallel to the retinal surface. 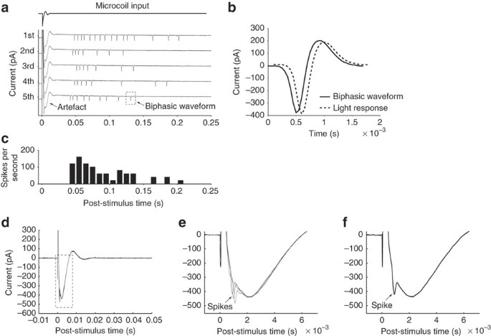Figure 4: μMS coil orientation alters neuronal response. (a) Ganglion cell responses to a single pulse of μMS (five repetitions); input to the microcoil is shown at top. Responses consisted of a prolonged stimulus artefact followed by a series of biphasic waveforms. (b) Overlay of light-evoked action potential and μMS-evoked biphasic waveform. Each trace is the average of five responses. Horizontal offset of the traces was utilized to facilitate comparison. (c) Peri-stimulus histogram of the firing rate for the five repetitions shown in (a). (Bin width: 10 ms). Stimulus pulse amplitude was 3 V and the main axis of the coil was oriented parallel to and 300 μm from the retinal surface. (d) Ganglion cell responses to a single μMS pulse when the main axis of coil was oriented perpendicular to retinal surface (overlay of five trials). (e) An expanded view of the responses; note three of the five traces elicited action potentials. (f) An expanded view of a single trial for which an action potential was elicited. Figure 4: μMS coil orientation alters neuronal response. ( a ) Ganglion cell responses to a single pulse of μMS (five repetitions); input to the microcoil is shown at top. Responses consisted of a prolonged stimulus artefact followed by a series of biphasic waveforms. ( b ) Overlay of light-evoked action potential and μMS-evoked biphasic waveform. Each trace is the average of five responses. Horizontal offset of the traces was utilized to facilitate comparison. ( c ) Peri-stimulus histogram of the firing rate for the five repetitions shown in ( a ). (Bin width: 10 ms). Stimulus pulse amplitude was 3 V and the main axis of the coil was oriented parallel to and 300 μm from the retinal surface. ( d ) Ganglion cell responses to a single μMS pulse when the main axis of coil was oriented perpendicular to retinal surface (overlay of five trials). ( e ) An expanded view of the responses; note three of the five traces elicited action potentials. ( f ) An expanded view of a single trial for which an action potential was elicited. Full size image Coil orientation influences neuronal responses In contrast to the burst responses elicited when the orientation of the coil was parallel to the retinal surface, the response to μMS consisted of only one or two spikes when the coil orientation was perpendicular to the retinal surface ( Fig. 4d–f ). The first spike always occurred within the stimulus artefact and its latency (Methods) ranged from 0.3–0.6 ms. Similar responses were observed in all 6 cells for which the coil was oriented perpendicularly. Changes to the amplitude of the μMS pulse altered the response to stimulation ( Fig. 5 ). In the parallel configuration, increases in the amplitude of the pulse elicited a larger number of spikes ( Fig. 5a , compare responses to amplitudes of 4 versus 6 volts). To examine the sensitivity to amplitude changes across the population of cells, the number of spikes elicited at each amplitude was averaged across five trials ( Fig. 5b ); average counts were then plotted as a function of stimulus amplitude. Lines connect individual points from the same cell. All cells tested in the parallel configuration ( n =6) exhibited an increase in the level of spiking with increased stimulation amplitude ( Fig. 5b ). Similarly, the responses arising from the perpendicular orientation were also sensitive to stimulus amplitude ( Fig. 5c ) ( n =6). However, because there were only 1 or 2 spikes elicited with this orientation, the increase in sensitivity was observed as an increased likelihood of eliciting the spike (or doublet). Increases in stimulus amplitude were also found to reduce the latency of elicited spikes ( Fig. 5d,e ). This reduction in latency occurred for both configurations (parallel: n =5/5; perpendicular: n =3/3). For the perpendicular configuration in which latencies were small to begin with, the decreases in latency were correspondingly small as well. In the parallel configuration, there was a small decrease in latency in all cells tested, but for two cells, the drop was >25 ms. Our results do not reveal the reason(s) for the large variability in latency shifts but it is possible that alternative, faster-acting mechanisms become activated at higher amplitude levels. 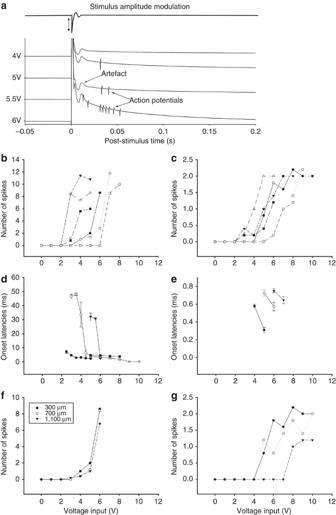Figure 5: Stimulus amplitude and coil-to-cell distance alter response properties. (a) Microcoil input (top trace) and ganglion cell response (bottom traces) to a series of increasing amplitude pulses (parallel-oriented coil). Amplitude levels range from 4 to 6 V. (b) Summary of responses to increasing amplitude stimulation for parallel orientation. Each point represents the average number of spikes elicited at the corresponding amplitude; lines connect all points from a given cell. (c) Summary of responses from perpendicular orientation. (d,e) The onset latencies of elicited spikes as a function of amplitude for stimulation in the parallel (d) and perpendicular (e) orientation. Bars represent standard errors (n=5). (f,g) Response sensitivity to location of the coil. Number of spikes is plotted as a function of stimulus amplitude for three different separations between coil and retina. At each separation, the number of spikes was averaged across five repetitions. (f) Parallel orientation of coil. (g) Perpendicular orientation of coil. Figure 5: Stimulus amplitude and coil-to-cell distance alter response properties. ( a ) Microcoil input (top trace) and ganglion cell response (bottom traces) to a series of increasing amplitude pulses (parallel-oriented coil). Amplitude levels range from 4 to 6 V. ( b ) Summary of responses to increasing amplitude stimulation for parallel orientation. Each point represents the average number of spikes elicited at the corresponding amplitude; lines connect all points from a given cell. ( c ) Summary of responses from perpendicular orientation. ( d , e ) The onset latencies of elicited spikes as a function of amplitude for stimulation in the parallel ( d ) and perpendicular ( e ) orientation. Bars represent standard errors ( n =5). ( f , g ) Response sensitivity to location of the coil. Number of spikes is plotted as a function of stimulus amplitude for three different separations between coil and retina. At each separation, the number of spikes was averaged across five repetitions. ( f ) Parallel orientation of coil. ( g ) Perpendicular orientation of coil. Full size image For each configuration, the sensitivity to stimulation was explored as the distance between the μMS coil and the targeted cell was varied ( Fig. 5f,g ). Similar to the previous experiment, the number of spikes elicited at each amplitude was determined for a fixed separation between coil and cell. The separation was then increased from 300 to 700 μm and then to 1,100 μm; at each increased separation, a new series of measurements was made. Responses to stimulation from both parallel and perpendicular orientations are shown in Fig. 5f,g , respectively. A slight decrease in sensitivity was observed as the coil was moved away from the cell for all 4 cells in which this experiment was run ( n =4); however, robust responses were observed even for separations of 1,100 μm. This suggests that μMS may create a fairly large zone of activation. Because the rate at which threshold increases for electric stimulation is proportional to the square of the distance between the cell and the electrode, our results also suggest that the sensitivity to distance is less for μMS than that of electric stimulation. There was one additional observation worth mentioning. At high stimulus amplitudes, the μMS pulse generated a 'disturbance' in the perfusion bath. The disturbance appeared as a transient flow of perfusion solution across the video monitor in which the cell and surrounding environment were observed ( Fig. 3c ). It is unlikely that this flow was necessary for activation to occur as there was no observed disturbance at lower stimulus amplitudes, even though spiking was elicited. Further, the latency of the first spike was <1 ms in one-half of the cells we tested ( n =6), strongly suggesting that activation was non-synaptic (that is, direct) in these cells. Therefore, even if a distal disturbance, outside the field view of the camera, activated neurons presynaptic to the ganglion cell, the delays associated with synaptic transmission would result in onset latency (for ganglion cell spiking) of greater than 1 ms. The increased flow did not alter the position of the cell, the position of the recording electrode or the impedance of the patch connection between the two, even at high amplitudes. This eliminates the possibility that responses arose from some form of mechanotransduction, (that is, movement of the patch electrode did not act as a mechanical stimulus). Nevertheless, we cannot rule out the possibility that, at high amplitudes, the transient change in flow rate influenced the responses. Although we did not investigate the source of this disturbance, it seems likely to arise from some form of mechanical resonance in the coil. The experiments conducted in this study represent an important first step in exploring the potential clinical applications of μMS. Computational simulations predicted that the coil design and range of stimulation parameters used here would generate an electric field that was sufficiently strong to activate neurons. Consistent with these findings, a series of electrophysiological experiments revealed that neural activity is elicited in response to μMS. Potential contributions from several non-magnetic factors including leaking electrical current, heating of tissue, and mechanical vibration were all eliminated allowing us to conclude that small magnetic fields can elicit action potentials. Because such coils are small enough to be implanted into both the cortex and deep subcortical nuclei, our results raise the possibility that μMS may be a viable alternative to existing DBS devices and other neural prosthetics. Previous studies of the retinal ganglion cell response to electric stimulation revealed two modes of activation: (1) direct activation of the ganglion cell and (2) indirect, or secondary activation resulting from activation of neurons presynaptic to the ganglion cell [5] , [27] . Each mode of activation has a distinct response signature: direct activation typically results in a single action potential with latency ≤1 ms, while the indirect response is more complex and typically consists of one or more bursts of spiking that have slower onset and persist for tens or hundreds of ms. Our results suggest that both modes of activation were also elicited by μMS: those neurons in close proximity to the (circular) end surfaces of the coil elicited one or two spikes only while those neurons along the cylindrical lengths of the coil exhibited bursts of spikes. Thus, our results also suggest that magnetic stimulation can elicit neuronal responses through at least two different modes of activation. Further, it is likely that the mode of activation is dependent on the location of the cell relative to the geometry of the coil: those ganglion cells close to the circular end surfaces of the coil were activated directly whereas those ganglion cells closer to the cylindrical lengths of the coil were activated secondary to activation of deeper (presynaptic) neurons. The mechanisms underlying activation are thought to be different for the two modes. Direct activation is thought to occur through rapid depolarization of the voltage-gated sodium channels in the proximal and distal portions of the axon. The mechanism underlying indirect activation is not known, but modelling studies suggest that as the slower acting voltage-gated calcium channels in the axon terminal [28] become activated, the ensuing inflow of calcium mediates an increased release of synaptic neurotransmitter. The temporal kinetics of the induced electric field from μMS was presumably the same at all locations and therefore it is somewhat surprising that responses to a given pulse were different for different locations around the coil. One possibility is that other mechanisms (that is, not ion channel kinetics) contribute to the response differences at different regions. Differences in the spatial properties of the induced electric field at the two locations ( Fig. 1 ) may have a role, although further work will be needed to determine the actual mechanism(s). Regardless of the exact mechanism of activation, the ability to generate both modes of activation may serve to enhance clinical outcomes. For example, methods that can selectively target presynaptic terminals may help to maximize the effectiveness of DBS stimulation [29] . In addition, the orientation of the μMS coil could be used to mitigate the side effects arising from unwanted axonal activation, that is, a primary side-effect of DBS therapy is the activation of adjacent tissue that result in the paresthesias [30] , [31] , [32] , [33] . Further enhancements to selectivity could arise from changes to the coil design, for example, lengthening the coil and reducing the diameter might help to further avoid the activation of axons. The responses to μMS exhibited similarities to the responses elicited by electric stimulation. For example, a larger number of spikes were elicited as the amplitude of the μMS pulse increased. In addition, the number of elicited spikes decreased as the distance between coil and cell increased, although the decrease in sensitivity for μMS was smaller than that for electric stimulation. These findings raise the possibility that the volume of activated neurons arising from a μMS coil could be considerably larger than that from conventional electrical stimulation devices. This may prove to be beneficial because chronic electric stimulation technologies lose efficacy with the formation of glial scars [34] , [35] , [36] , [37] , [38] and μMS activation may still be effective even for the largest size scars. The simulations we performed suggest that sensitivity to distance can be modulated by changes in the coil geometry (and/or the parameters of stimulation) and further testing will be needed to determine how well the region of activation can be tailored to the needs of specific applications. Although the current study is prefaced on the potential clinical applications for the μMS coils, there is also a potential for this technology to be utilized in experimental settings. Namely, because the technology is inherently MRI compatible, it could be used as an alternative to TMS, FES, or peripheral electrical stimulation during imaging studies. In addition, because μMS coils can be used in both in vivo and in vitro preparations, there are opportunities to use these devices to investigate the mechanism of action of DBS, FES, or TMS. Finally, although we have demonstrated computationally and empirically that μMS can modulate neuronal activities, further studies are needed to understand the relationship between the parameters of magnetic stimulation and neuronal activation as well as the effects on μMS on different neuronal elements (for example, presynaptic, postsynaptic, soma and axonal) and the spatial characteristics of μMS fields in different brain tissues. Coil calculations A model of a coil with metal terminals was positioned inside a homogeneous volume conductor representing the saline solution or the retinal tissue. The model was implemented using FEM simulations to determine whether such small coils could generate electric fields strong enough to evoke action potentials in neuronal tissue, provided the coils were positioned close to excitable cells. All of the electromagnetic quantities introduced in this work are summarized in Table 1 . An inductor is the ideal magnetic field generator, and it stores the magnetic field energy W generated by the supplied electric current i . Simulations were performed by considering low frequencies (that is, where l is the maximum dimension of the object and f 0 is the maximum current frequency) and ignoring the contribution of the displacement currents (that is, ). The optimal μMS coil is an inductor with magnetic energy W : where A is the magnetic potential, and the curl is the magnetic flux density (that is, B = × A ). The portion of energy W lost reduces the Q-factor or efficiency and the inductance of the coil. Part of the magnetic energy W in equation (1) is therefore available to elicit neuronal activity. The electric fields and magnetic flux densities were found by solving numerically the following magnetostatics equation [39] : where σ is the electrical conductivity expressed in S / m . Table 1 Nomenclature, dimensions and constants used in the FEM simulations. Full size table The induced currents and electric fields in the tissue are expressed by Faraday's law: where Φ is the scalar potential. Let us now consider the following cylindrical coordinates ( r , z , φ ), where the coil is in the rz plane (that is, ( r , z 0 , φ )) and each turn of the coil has coordinates r i and φ [0;2 π ]. We assumed that Φ = 0 (ref. 40 ), because in an unbounded medium, Φ is only due to free charges and no such sources are present. Furthermore, we consider the frequency domain by assuming time harmonic fields with angular frequency ω and we will perform simulations with the maximum frequency (70 kHz) of the class D amplifier used in the experiments, as the pulse can be represented as 1/2 of a sinusoidal/cosinusoidal function. The induced electric fields E = − jω A (or equation (3) transformed in frequency domain) were found by solving the following quasistatic equation [39] : where J e is the external current, u φ is the unit vector in the φ -direction and each turn of the coil, approximated by a circle with radius r and potential V r , has an electric current amplitude derived from: FEM numerical simulations were conducted to study the microscopic magnetic flux density generated by the MEMS microinductor ( Fig. 6 ). The FEM simulations were performed in Multiphysics 4.2a with the AC/DC module (COMSOL, Burlington MA, USA) using the emqa model or the electromagnetic quasi-static approximation. 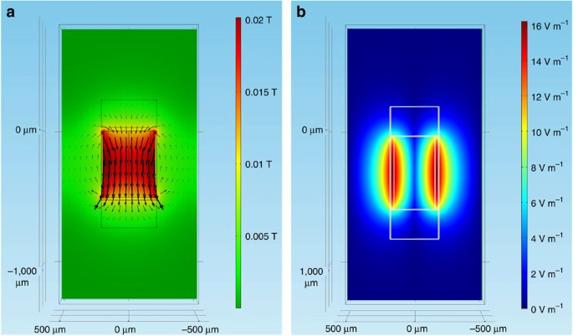Figure 6: Magnetic and electric field distributions on theyz-plane. (a) The magnetic field (in Tesla) distribution on theyz-plane (x=0) μm using the same coordinate system as inFig. 1. (b) The magnitude of the electric field (V m−1) induced in and around the microcoil. The colourmap shows the current density at each point of the plane, and the lines uniformly sample the magnetic flux density in 20 bins. Figure 6: Magnetic and electric field distributions on the yz -plane. ( a ) The magnetic field (in Tesla) distribution on the yz -plane ( x =0) μm using the same coordinate system as in Fig. 1 . ( b ) The magnitude of the electric field (V m −1 ) induced in and around the microcoil. The colourmap shows the current density at each point of the plane, and the lines uniformly sample the magnetic flux density in 20 bins. Full size image The model of induced electric fields was solved for the magnetic vector potential A in equation (4). There were no weak constraints, and all constraints were ideal. The overall geometry consisted of a cylinder of 3.0 mm in radius and 3.0 mm in height and was chosen to study the induced electric field around the coil which contained four different types of objects: a solenoid coil, two terminals, a quartz core and physiological solution. The solenoid consisted of 21 turns (rings) and was 500 μm in height and 500 μm in internal diameter as well as a 5μm×10 μm trace section. The terminals were two cylinders of 200 μm in radius and 200 μm in height. The quartz core consisted of 500 μm diameter and 500 μm in height on top and on the bottom copper terminals. The physiological solution was a cylinder of 3.0 mm in radius and 3.0 mm in height. Table 1 describes the material properties of the coil and the surrounding physiological solution/tissue and the constant values used in the simulations. Further details are provided in Supplementary Methods . Preparation and testing of μMS coils Coil assembly is described in Supplementary Methods . Assembled coils were manually coated with a xylene-based dielectric varnish (Gardner Bender, Milwaukee, WI, USA). This hand operation resulted in a non-uniform coating of dielectric as well as an irregular (non-smooth) outer surface. Because the dielectric was opaque to the infrared illumination system used during in vitro experiments, it was necessary to establish the approximate location of the coil relative to the outer boundaries of the dielectric-coated assembly (typically ~200 μm). Because the dielectric-coated coil assembly was much larger than the field of view, it was not trivial to determine the height of the coil above the retinal surface during an experiment. Preliminary measurements under bright illumination revealed the position of the coil within the dielectric and were also used to determine the exact outer limits for each (coated) coil assembly. In this manner, the bottom edge of the coil assembly was determined relative to a focal point at or near the top surface of the assembly, and the height of the coil above the retinal surface could be reasonably estimated. In this manner, the distance from the retinal preparation to the closest edge of the coil could be reliably controlled and was set to 100 μm in most experiments. Although the exact thickness of the dielectric was difficult to ascertain, the approximate thickness was 200 μm and, therefore, the coil to retina distance is listed as 300 μm. We estimate the actual variability of the dielectric thickness to be ±50 μm. The increases in distance associated with the experiments of Fig. 5 were obtained via a 400 (or 800)-μm translation in the z -direction using the micromanipulator. The μMS coil assemblies were tested before and after each experiment to ensure that there was no leakage of current. If present, such currents could have produced the observed neural activity. The coils were submerged in physiological solution (0.9% NaCl) and the impedance between one of the coil terminals and an electrode immersed in the physiological solution was measured before and after each electrophysiological experiment. Impedances above 5 MΩ were considered indicative of adequate insulation. Liquid Teflon was selected because of its high dielectric strength (>100 V μm −1 ), and the 5 MΩ value was based on the fact that Teflon has very low conductivity (typically 10 −23 S m −1 ) and that the tester was not able to reliably measure high impedances as it had a low dynamic range. μMS drive The output of a function generator (AFG3021B, Tektronix, Beaverton, OR, USA) was connected to a 1,000 W audio amplifier (PB717X, Pyramid, Brooklyn, NY, USA) with a bandwidth of 70 kHz. Positive and negative pulses were created alternately by the function generator at a rate of 1 pulse per second. Pulse amplitudes ranged from 0–10 V in steps of 0.5 V and the rate of increase of the leading edge was 18 ns V −1 ; the decrease of the trailing edge occurred at an equal rate. The output of the amplifier consisted of a sharp peak followed by a damped cosine waveform (monitored with a DPO3012 oscilloscope (Tektronix, Beaverton, OR)). The peak had maximum amplitudes ranging from 0–46 V (4.6 V V −1 ) with leading/trailing edge slopes of 80 ns V −1 . Its duration was ~20 μs. The amplitude of the damped sinusoid was smaller than the peak and ranged from 0–12 V; its duration was ~12 ms. Electrophysiology The extraction and mounting of the rabbit retina as well as the use of cell-attached patch clamp recordings followed well-established procedures [25] and are described in detail in Supplementary Methods . Patch pipettes were used to make small holes in the inner limiting membrane, and ganglion cells with large somata were targeted under visual control ( Fig. 3c ). Spiking was recorded with a cell-attached patch electrode (4–8 MΩ). Full-field light stimuli were used to determine whether an appropriate patch seal had been established and also to confirm that the cell was functioning normally; only those cells that generated spiking responses to light were tested with μMS. The μMS coil assembly was fixed in the micromanipulator such that the main axis of the coil was oriented either parallel or perpendicular to the retinal surface ( Fig. 3a,b ). The coil assembly was lowered into the bath until its bottom edge was 100 μm above the retinal surface; this corresponded to a coil height of ~300 μm. Five repeats were performed for each parameter set, that is, every time a parameter was changed. Data analysis Raw waveforms were recorded at a sample rate of 20 kHz and processed with custom software written in MATLAB. Each elicited waveform contained an electrical artifact arising from the μMS pulse; the artefact lasted ~20 ms and was nearly identical for trials with identical stimulus conditions. Many elicited responses also contained a series of action potentials (spikes); these were confirmed as spikes by comparing them to those spikes elicited in response to light stimuli (Results). The timing of individual spikes was determined with a 'matched filter'—the average light-elicited spike was cross-correlated with the response waveform; peaks in the cross correlation were used to assign timing of individual action potentials. How to cite this article: Bonmassar, G. et al . Microscopic magnetic stimulation of neural tissue. Nat. Commun. 3:921 doi: 10.1038/ncomms1914 (2012).